Quantitative characterization of nanoscale polycrystalline magnets with electron magnetic circular dichroism Electron magnetic circular dichroism (EMCD) allows the quantitative, element-selective determination of spin and orbital magnetic moments, similar to its well-established X-ray counterpart, X-ray magnetic circular dichroism (XMCD). As an advantage over XMCD, EMCD measurements are made using transmission electron microscopes, which are routinely operated at sub-nanometre resolution, thereby potentially allowing nanometre magnetic characterization. However, because of the low intensity of the EMCD signal, it has not yet been possible to obtain quantitative information from EMCD signals at the nanoscale. Here we demonstrate a new approach to EMCD measurements that considerably enhances the outreach of the technique. The statistical analysis introduced here yields robust quantitative EMCD signals. Moreover, we demonstrate that quantitative magnetic information can be routinely obtained using electron beams of only a few nanometres in diameter without imposing any restriction regarding the crystalline order of the specimen. Modern synchrotron X-ray sources, delivering intense radiation with well-defined polarization, have provided insight into the magnetic aspects of solids [1] . The usefulness of synchrotron X-rays in magnetism can be attributed to the discovery of an important phenomenon: X-ray magnetic circular dichroism (XMCD) [2] , [3] , [4] . XMCD originates from the dependence of the absorption cross-section on the sample magnetization with respect to the photon helicity. Spin and orbital magnetic moments can be quantitatively determined in an element-specific manner using a simple integration of the XMCD spectra employing sum rules [5] , [6] . An analogue to XMCD is the electron magnetic circular dichroism (EMCD) technique, in which electrons are transmitted through a magnetic sample in a transmission electron microscope (TEM) [7] , [8] . Electron energy loss spectroscopy (EELS) measured at core levels can then be employed to extract element-selective magnetic information. The possible existence of EMCD was first outlined in 2003 (ref. 7 ) using methods reminiscent of symmetry-selected EELS [9] . Recent theoretical and experimental progress in the EMCD technique led to improvements in its spatial resolution [10] , [11] and theoretical understanding [12] , [13] , [14] , [15] , [16] and provided the first quantitative studies [17] , [18] , [19] of spin and orbital magnetic moments. Owing to the very short de Broglie wavelength of the high-energy electrons, TEM offers a much higher spatial resolution than that currently obtainable with XMCD. However, high-resolution quantitative EMCD has never been achieved because of its inherent low net signal strength. Being measured at core-level edges, the EMCD signal strength exhibits a power-law decay as a function of energy loss. Another challenge is the necessity to measure EMCD at diffraction angles that do not coincide with Bragg spots in the diffraction plane, which reduces the signal strength even further. Moreover, beam and sample instabilities, coupled to a potential damage of the sample by an intense electron beam, limit the acquisition time. In most experiments performed to date, a large beam current was used in an optimized geometry—namely, the 2-beam [8] , [14] , [17] , [20] , [21] or 3-beam [11] , [17] , [19] , [22] Bragg condition—which in turn implies a demand for a single-crystalline specimen in a precise and stable orientation. In this work, rather than optimizing the signal-to-noise ratio (SNR) in a fixed geometry—a procedure that is inherently prone to beam damage and stability issues—we rapidly collect a large number of independent spectra and introduce a new statistical technique for the analysis, efficiently overcoming the aforementioned restrictions and reducing the lateral resolution of quantitative EMCD to the nanometre range. We demonstrate the power of the technique by analysing a polycrystalline iron sample. Theoretical background The approach proposed in this paper has been inspired by simulated distributions of dichroic signals in the diffraction plane [12] , [15] that suggest that EMCD is present almost everywhere in the diffraction plane, despite non-trivial variations in strength and sign. The underlying reason involves the decomposition of the inelastic transition matrix elements (mixed dynamic form factor—MDFF) in a dipole approximation to a linear combination of non-magnetic and magnetic terms, including their anisotropies [15] . In a material with a cubic crystal structure, such as bcc iron, the anisotropic terms are negligible, and a simple expression for the MDFF S ( q , q′ ,E) remains: where q , q ′ are momentum transfer vectors, E is the energy loss and N ( E ), M z ( E ) are the white-line non-magnetic signal and magnetic EMCD signal, respectively. In this equation, it has been assumed that the sample is magnetically saturated along the z axis in the magnetic field of the objective lens. At an arbitrary relative orientation of the crystalline axes, incoming beam and detector, the scattering cross-section will be a weighted sum of these terms: with coefficients A (Ω) and B (Ω) that depend on the diffraction angle Ω. Consequently, we establish that for a bcc-iron polycrystalline sample with sufficiently large grains, every spectrum is a linear combination of a white-line non-magnetic signal N ( E ) and a magnetic EMCD signal M z (E), albeit with a priori unknown coefficients A (Ω) and B (Ω). Experiment Rather than measuring a few energy-filtered diffraction patterns [17] , [20] or a few spectra [21] , [22] in a well-defined scattering geometry, we acquire a large number—up to several hundred—of spectra in a random alignment of incoming beam and detector orientations with respect to the lattice axes of an illuminated grain. The acquired large data set forms the starting point for our statistical procedure leading to the extraction of the EMCD spectrum. In the measurement, we use an ultra-high-voltage (1 MV) electron beam to significantly reduce the effect of multiple scattering, which could otherwise distort the EMCD signal [18] . Our theoretical simulations indicate that the net EMCD signal at an accelerating voltage [23] of 1 MV is ~20% larger than that obtained at 200 kV for a specimen thickness between 25 and 40 nm (for details, see Supplementary Fig. 1 ). The studied sample is a fine-grain polycrystalline bcc iron film ( Fig. 1b ) with a thickness of ~30 nm. A schematic diagram of our experimental setup is presented in Fig. 1a . The same acquisition procedure was repeated three times independently on different areas of the sample, yielding three independent data sets. 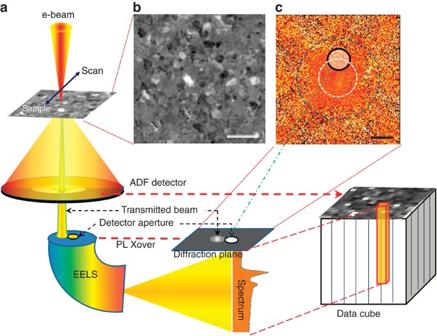Figure 1: Schematics of the proposed scanning-mode measurement of EMCD. (a) Schematic drawing of the experimental setup and the data obtained (ADF: annular dark field, PL: projector lens). The detector aperture is placed at the PL cross-over position. In the present STEM mode, the PL cross-over position is on the diffraction plane. (b) A TEM image of the investigated polycrystalline iron film. Scale bar, 50 nm. (c) Calculated EMCD signal intensity distribution of a polycrystalline iron film in the diffraction plane. The highlighted area indicates the measured area covered by the detector entrance aperture. The detector entrance aperture (solid circle) is located at the position of 0.4 g(110)away from the origin, and its diameter is 0.5 g(110). The white broken circle represents the possible aperture centre positions in the diffraction plane and blue broken circle corresponds to g(110)ring position for comparison. Scale bar, 2 nm−1. The minimum (black) and maximum (white) EMCD values range from −3 to +3%. Figure 1: Schematics of the proposed scanning-mode measurement of EMCD. ( a ) Schematic drawing of the experimental setup and the data obtained (ADF: annular dark field, PL: projector lens). The detector aperture is placed at the PL cross-over position. In the present STEM mode, the PL cross-over position is on the diffraction plane. ( b ) A TEM image of the investigated polycrystalline iron film. Scale bar, 50 nm. ( c ) Calculated EMCD signal intensity distribution of a polycrystalline iron film in the diffraction plane. The highlighted area indicates the measured area covered by the detector entrance aperture. The detector entrance aperture (solid circle) is located at the position of 0.4 g (110) away from the origin, and its diameter is 0.5 g (110) . The white broken circle represents the possible aperture centre positions in the diffraction plane and blue broken circle corresponds to g (110) ring position for comparison. Scale bar, 2 nm −1 . The minimum (black) and maximum (white) EMCD values range from −3 to +3%. Full size image Extraction of the EMCD spectrum After pre-processing the 225 measured spectra (see Methods), we calculated a difference spectrum for every pair of the spectra present in the data set, which yielded a total of 25,200 difference spectra per data set. All the difference spectra were subsequently examined one-by-one for the presence of an EMCD signal using criteria that probe the relative signs of intensity around the L 3 and L 2 edges: where represents the EMCD signal intensity integrated over the Fe-L 3 peak region and I Δ σ (at L 3 peak) denotes the EMCD signal value at the L 3 peak position. All the difference spectra that passed our selection criteria were first aligned in sign such that the L 3 signal was positive and then summed. Approximately 20–25% of pairs out of the entire set of pairs always displayed signs of the EMCD signal and thus passed our selection criteria. Furthermore, we applied a low-pass filter to obtain EMCD signals that are sufficiently smooth for quantitative analysis (see below). The final summed signal intensities and profiles for the three data sets were nearly identical (see Fig. 2b ). Minor differences were observed in the pre-edge and post-edge background regions, which were related to varying fluctuations between individual data sets. These differences can be attributed to inaccuracies in the extraction of the power-law background signal, which is caused by extrapolation from a noisy pre-edge signal. 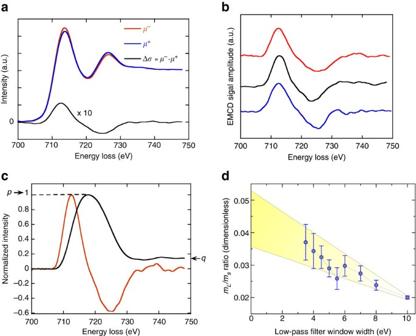Figure 2:Representative EELS and EMCD spectra. The representative spectra are measured on a fine-grain polycrystalline iron film by STEM–EELS at an accelerating voltage of 1 MV. A 5-eV low-pass filter was applied to the original spectra fora–cbelow. (a) A pair of Fe-L2,3EELS spectra (μ+and μ−) extracted from the data set and their difference spectrum (EMCD signal) Δσ=μ−−μ+. (b) EMCD signals extracted from the three independent data sets of different areas of the sample, plotted separately in red, black and blue, respectively. (c) The averaged EMCD signal (red curve) and its cumulative sum (black curve), which is required to apply the sum rule13,14.qis an energy integral of the EMCD signal over both edges, andpis an energy integral over the L3edge only. Without loss of generality, we can rescale the integral of the EMCD signal such thatp=1, as indicated, whereupon the orbital to magnetic moment ratiomL/mSis a function ofqonly, allowing an easy visual comparison of the energy integrals in the post-edge region. (d) Plot of themL/mSratio estimated by the sum rule as a function of the window width of the low-pass filter used for data smoothing. The error bars were estimated from the statistical fluctuation ofq. The shaded area was bounded by linear regression lines (grey solid lines) of the lower and upper bound values. The relation is linearly extrapolated to zero window width, and the netmL/mSis derived to be 0.0429±0.0075. Figure 2: Representative EELS and EMCD spectra . The representative spectra are measured on a fine-grain polycrystalline iron film by STEM–EELS at an accelerating voltage of 1 MV. A 5-eV low-pass filter was applied to the original spectra for a – c below. ( a ) A pair of Fe-L 2,3 EELS spectra (μ + and μ − ) extracted from the data set and their difference spectrum (EMCD signal) Δ σ = μ − − μ + . ( b ) EMCD signals extracted from the three independent data sets of different areas of the sample, plotted separately in red, black and blue, respectively. ( c ) The averaged EMCD signal (red curve) and its cumulative sum (black curve), which is required to apply the sum rule [13] , [14] . q is an energy integral of the EMCD signal over both edges, and p is an energy integral over the L 3 edge only. Without loss of generality, we can rescale the integral of the EMCD signal such that p =1, as indicated, whereupon the orbital to magnetic moment ratio m L / m S is a function of q only, allowing an easy visual comparison of the energy integrals in the post-edge region. ( d ) Plot of the m L / m S ratio estimated by the sum rule as a function of the window width of the low-pass filter used for data smoothing. The error bars were estimated from the statistical fluctuation of q . The shaded area was bounded by linear regression lines (grey solid lines) of the lower and upper bound values. The relation is linearly extrapolated to zero window width, and the net m L / m S is derived to be 0.0429±0.0075. Full size image We averaged the three accumulated EMCD signals to obtain the final EMCD spectrum, which is presented in Fig. 2c . The EMCD signal intensity fraction was estimated to be 2–2.3% of the Fe-L 2,3 signal intensity ( Fig. 2a ), which is consistent with the theoretical estimate (see Supplementary Fig. 1 ). The final EMCD signal is a result of averaging over ~15,000 different spectra and was thus observed to be statistically robust. Quantitative analysis After extraction of an EMCD signal with a good SNR, the EMCD sum rules were applied to the signal to evaluate the orbital moment/spin moment ratio, given by [13] , [14] : where q is an energy integral of the EMCD spectrum Δ σ ( E ) over both edges and p is an energy integral over the L 3 edge only. Without loss of generality, we can rescale the EMCD spectrum or its integral such that p =1 ( Fig. 2c ). Thus, the orbital to magnetic moment ratio m L / m S becomes a function of q only. The application of the low-pass filter can possibly lead to overlap and cancellation of the EMCD signals of the L 3 and L 2 peaks, which could equally reduce the magnitude of both peaks and consequently enhance the effect of their difference. Moreover, the application of the low-pass filter can affect the post-edge normalization [24] . The latter could alter the m L /m S ratio that is determined using the sum rules. The m L / m S ratio was hence plotted as a function of the low-pass filter window width and extrapolated to zero window width, as illustrated in Fig. 2d . The error bar of the individual data points represents the fluctuation of q in the post-edge region between 740 and 750 eV. By linear extrapolation to zero filter width, we finally obtained m L / m S =0.0429±0.0075, which is in good agreement with the value obtained by XMCD for bcc iron—that is, 0.043 (ref. 4 ). Our result represents the first quantitative EMCD detection performed on a polycrystalline film. The measurements were carried out using EELS spectral imaging with an ultra-high-voltage scanning transmission electron microscope (STEM), the JEM 1000 K RS of the Nagoya University. The STEM was operated at 1 MV and equipped with an equivalent Gatan Image Filter Quantum, which is specially designed for this accelerating voltage. The sample was heated to 200 °C during the experiment so that measurements were contamination-free. The full-width at half-maximum of the zero-loss peak was ~2.6 eV because the beam current had been increased to ensure an increase in spectral counts. The electron beam was focused to ~5 nm and scanned 15 × 15 pixels on the sample with a scan step of 20 nm. This configuration guaranteed that the electron beam illuminated random grains, typically one or a few grains at each scanned position. The approximate convergence semiangle of the probe was ~1 mrad. EELS spectra were recorded with a dispersion of 0.5 eV per channel, exposure time of 30 s for each spot and a collection semiangle of ~1 mrad, where 1 mrad~0.23 g (110) ~1.12 nm −1 . The detector aperture was located at a position next to the transmitted beam in the diffraction plane to avoid including the intense transmitted beam ( Fig. 1a ). Under these conditions, the Fe-L 3 peak intensities ranged between 8,000 and 12,000 counts per spectrum. The same experiment was repeated independently for three different areas. We stress that, whereas a 5-nm nanoprobe was used, the spectral differences were computed from the entire data stack, rendering the effectively sampled area to be of the order of 100 nm. This area could be reduced by changing the scanning pattern, provided that sufficiently random orientations were included in each data set. Although the measured m L /m S ratio corresponds well to the value known from XMCD measurements, it is imperative to analyse the robustness of our statistical scheme. Several error sources that affect the statistical extraction of the EMCD signal can be identified. The main error source of our extraction method of the EMCD spectrum stems from the imperfection of the employed detectors: the recorded raw spectra may include significant fractions of systematic errors, which originate from instrumental instabilities and concomitant intrinsic limitations in addition to the statistical random noise. For the reasons stated above, we observed that conventional statistical signal extraction methods such as the one based on multivariate curve resolution technique [24] were not efficient, and it was essential that the data should be first sorted to select only the data sets containing significant signal levels based on the present selection criteria (equation (3)) applied to the difference spectra. To eliminate the possibility that our procedure might lead to a fake EMCD-like signal profile extracted from a random noisy data array, we performed an equivalent set of measurements on an antiferromagnetic NiO film, in which no EMCD signal was expected due to the cancellation of magnetic signals from symmetrically equivalent atoms with antiparallel moments. The sample was a NiO polycrystalline film (grain size ~30 nm, film thickness ~30 nm), and the measurements were performed under the same conditions (at 165 °C—that is, below the Néel temperature) as for the bcc iron film. Subsequently, the same data processing was applied to the Ni L 2,3 white-line spectra. The noise level was estimated by taking the square-root of the sum of squares of the difference spectra between the raw and median filtered (averaged over every 10 channels) spectra divided by the number of channels used for the analysis. Then, the SNR was estimated by dividing the intensity at the L 3 peak position of the averaged EMCD signal by the noise level. The estimated SNR was 2–3 for bcc iron, whereas it was <0.5 for NiO. The averaged signal extracted from the NiO data actually was observed to exhibit a bimodal EMCD-like profile; however, the profile significantly varied upon changing the integration width for the first selection criterion, and the q -value from the sum rule was sometimes positive and sometimes negative, without a clear trend with respect to the filter width. The bimodal profile is a result of the selection requirements (equation (3)), which extract all EMCD-like difference-spectra naturally occurring in the set of completely random difference spectra. However, the signal profiles extracted from the iron film exhibited a stable feature. The situation can be best observed from the overlaid typical difference spectra passing the selection criteria for the two cases, as shown in the upper panels of Fig. 3 . For the iron film, one can clearly recognize an approximate EMCD signal profile, whereas for the NiO film, the spectra visually differ only slightly from random noise. 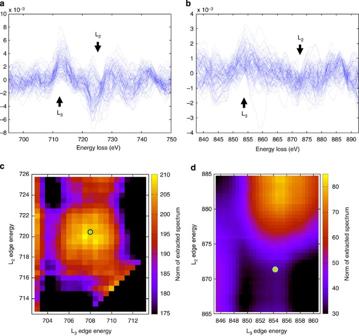Figure 3: Statistical significance tests of the extracted EMCD signals. The tests are applied to ferromagnetic and non-ferromagnetic samples. (a) Example of difference spectra for a polycrystalline bcc Iron film. A random EELS spectrum was selected from a data set, and all 224 difference spectra were tested using our selection criteria (see Methods). Only spectra that passed the criteria are shown, after being aligned in sign. (b) Same asabut for a polycrystalline NiO film. The arrows indicate the L3and L2peak positions of the raw spectra. Note the different scale of the vertical axes relative to the post-edge normalized spectra, considering that all raw spectra were normalized to 1 in the post-edge region. (c) Maps of the norm of the extracted averaged spectrum as a function of the L2and L3edge energies for the polycrystalline bcc iron sample (see Discussion). (d) Same ascbut for the antiferromagnetic NiO film. The green circles indicate experimental edge energies. The integration range is ±5 eV around the edge energy, and the median filter width is 7 eV. Both results originate from a data set of 225 spectra, post-edge normalized to one. Note again the different scales of the norms. Figure 3: Statistical significance tests of the extracted EMCD signals. The tests are applied to ferromagnetic and non-ferromagnetic samples. ( a ) Example of difference spectra for a polycrystalline bcc Iron film. A random EELS spectrum was selected from a data set, and all 224 difference spectra were tested using our selection criteria (see Methods). Only spectra that passed the criteria are shown, after being aligned in sign. ( b ) Same as a but for a polycrystalline NiO film. The arrows indicate the L 3 and L 2 peak positions of the raw spectra. Note the different scale of the vertical axes relative to the post-edge normalized spectra, considering that all raw spectra were normalized to 1 in the post-edge region. ( c ) Maps of the norm of the extracted averaged spectrum as a function of the L 2 and L 3 edge energies for the polycrystalline bcc iron sample (see Discussion). ( d ) Same as c but for the antiferromagnetic NiO film. The green circles indicate experimental edge energies. The integration range is ±5 eV around the edge energy, and the median filter width is 7 eV. Both results originate from a data set of 225 spectra, post-edge normalized to one. Note again the different scales of the norms. Full size image As an additional test of the statistical robustness of the polycrystalline iron EMCD result, in contrast to the averaged NiO signals originating from noise, we varied the L 2,3 peak energies in the neighbourhood of their experimental values in our extraction procedure. At every combination of the L 2,3 edge energies, an averaged EMCD-like signal was constructed. For every extracted signal, we calculated its norm as a sum of squares within the edge integration intervals. If a true EMCD signal was present in the data, this sum of squares would have a local maximum near the physically correct values of the edge energies. The bottom panels of Fig. 3 present maps of the norms calculated for a median filter of 7 eV and an integration range ±5 eV around the assumed peak energies, with the L 3 energy as its abscissa and the L 2 energy as its ordinate. A green circle denotes the position of the L 3 /L 2 peak energies, in which the experimental white-line spectra exhibit maximal counts. The striking difference between the two plots clearly demonstrates the validity of our method. The polycrystalline iron data reveal a distinct peak around the expected values of the edge energies, with a maximum within 1 eV from the experimental values. Conversely, the NiO spectra do not exhibit any such feature around the expected edge energies. In summary, we conclude that the method introduced in this paper leads to statistically significant EMCD spectra. Consequently, our approach allows quantitative EMCD studies of non-single-crystalline samples on the nanoscale and hence paves the way for a new era of application of EMCD experiments in the field of nano-magnetism. Sample fabrication A 30-nm-thick bcc iron layer and a 3-nm-thick Al cap layer (to prevent the oxidation of Fe) were deposited on 50-nm-thick Si 3 N 4 membranes by thermal evaporation in an ultra-high vacuum molecular beam epitaxy system. The thicknesses are controlled using calibrated quartz microbalances. Although no measurement (such as atomic force microscopy) that quantifies the thickness variations was performed, we estimate an upper limit for the thickness variations of the studied polycrystalline films of 1 nm, which corresponds to the relative thickness fluctuations of ~3% and ensures that no significant spectral intensity variation due to film thickness variation is expected. No ex situ or in situ preparation/cleaning was applied to the Si 3 N 4 membranes before the deposition. The membranes were kept at room temperature during the deposition. The disordered structure of the membranes (nanocrystalline or amorphous) led to a polycrystalline morphology of the metallic Fe/Al films. Air exposure after the deposition oxidized the Al cap layer to a depth of 1.5–2 nm. As the Al layer was 3-nm thick, a closed AlO x layer was maintained even in the presence of surface roughness (likely for a polycrystalline film). Some metallic Al may remain at the interface to the iron film. The approximate grain size was ~30 nm, which is comparable to the thickness of the iron layer ( Fig. 1b ). As oxidation of the iron film could have substantial effects on the intensity ratio of the L 3 and L 2 edges [25] , the film was examined with EELS to probe whether any oxidation of the iron occurred before or after the EMCD measurements using the fact that the oxygen K edge can be easily distinguished between aluminium and iron oxides. Nevertheless, no iron oxides were observed within the detection limit of EELS (<1 at %). The NiO sample used here was a standard reference sample supplied by Gatan Inc. and was prepared in the following manner: a thin polycrystalline Ni film was first prepared by sputtering Ni on a cleaved rock salt crystal. The polycrystalline film was subsequently floated off and mounted on a copper grid. The NiO film was then prepared by heating the metal film already supported on grids in air. Data processing The obtained spectral image data cubes were first treated by applying the ‘SI/Align by Peak’ and ‘Volume/Remove X-rays’ menu commands of the Gatan DigitalMicrograph software to align the drifted peak positions and remove X-ray spikes (very bright/dark spots). We then applied the pre-edge background subtraction to extract the Fe-L 2,3 peaks, after which we applied a low-pass filter with a window width that was variable from 3.5 to 10 eV. The filter acts by replacing the value in a given spectrum channel by the average number of counts per channel in an interval with a specified width and centred on the channel in question. We did not apply the Fourier-ratio deconvolution to remove the plural scattering effect because the plasmon peak-to-zero loss peak intensity ratio was <6%, therefore causing only a negligible difference to the final m L / m S ratio within the experimental accuracy [18] . The reduced size of the error attributed to the multiple scattering is another advantage of using a megavolt-STEM in addition to the improved strength of the EMCD signal compared with lower acceleration voltages, as discussed previously. Each measured spectrum was normalized by scaling the post-edge intensity integrated over the range 740–750 eV to one. The effect of this normalization on the quantitative analysis was discussed in a previous study [24] . In the first step, we examined the difference spectra for all pairs of the spectra in the data set. As described above, each spectrum can be considered as consisting of two components, a magnetic one (the EMCD) and a non-magnetic one. When a spectrum is acquired in a random orientation, the weight of each component is also random; however, once the spectra are background-subtracted and normalized post-edge (where the magnetic component is always zero), the non-magnetic component will be identical and will therefore be eliminated by taking the difference spectrum. Despite the noise and error propagation during the background subtraction and normalization, some (20–25%) difference spectra exhibited an EMCD signal, while others did not or were too noisy. All the difference spectra were filtered by selecting only those that satisfied the selection criteria (equation (3)); thus, we ensured that we were preferentially selecting the bimodal spectral features characteristic of the EMCD signals. We discarded the spectra that did not exhibit the EMCD signature. The selected subset (~5,000 difference spectra) originated from >100 independent raw spectra among the entire set of 225 spectra, which ensures that the statistical noise is reduced by a factor of 10 compared with the average noise of individual raw spectra. A cumulative sum was subsequently constructed from every EMCD spectrum extracted with various filter widths (see Fig. 2c for the 5-eV window width). The minimal and maximal q were extracted from the post-edge region between 740 and 750 eV energy loss, from which the minimal and maximal m L / m S were calculated. The m L / m S values with error bars are plotted as the middle points of these upper and lower bounds in Fig. 2d . The shaded area is bounded by linear regression lines (grey solid lines) at the lower and upper bound values. The final m L / m S was evaluated to be the intercept of the linear regression line (grey broken line) of the middle points +/− half of the interval defined by the intercepts of the bound lines. Simulations A bcc iron supercell of 4 × 4 × 18 lattice dimensions (~1 × 1 × 5 nm) containing 576 iron atoms was melted, annealed and slowly cooled in accordance with classical molecular dynamics and considering the interatomic potential proposed by Mendelev et al. [26] The procedure was repeated many times and, in some cases, we obtained a structure model with several crystalline grains with different orientations ( Supplementary Fig. 2a ). A representative structure model was used in our proof-of-concept simulations. The corresponding electron diffraction pattern is presented in Supplementary Fig. 2b . We calculated the electronic structure of this model structure using density functional theory and estimated an average magnetization of 2.19 μ B per atom. For calculations of the dynamical diffraction, this structure model was periodically repeated in x , y dimensions and illuminated by a plane wave. The calculated Fe-L 3 edge energy-filtered diffraction pattern of the magnetic signal along the z direction [16] is presented in Fig. 1c and Supplementary Fig. 2c . Approximately 600 beams were considered in the simulation [12] , [27] . How to cite this article: Muto, S. et al. Quantitative characterization of nanoscale polycrystalline magnets with electron magnetic circular dichroism. Nat. Commun. 5:3138 doi: 10.1038/ncomms4138 (2014).